Atomic transistors based on seamless lateral metal-semiconductor junctions with a sub-1-nm transfer length The edge-to-edge connected metal-semiconductor junction (MSJ) for two-dimensional (2D) transistors has the potential to reduce the contact length while improving the performance of the devices. However, typical 2D materials are thermally and chemically unstable, which impedes the reproducible achievement of high-quality edge contacts. Here we present a scalable synthetic strategy to fabricate low-resistance edge contacts to atomic transistors using a thermally stable 2D metal, PtTe 2 . The use of PtTe 2 as an epitaxial template enables the lateral growth of monolayer MoS 2 to achieve a PtTe 2 -MoS 2 MSJ with the thinnest possible, seamless atomic interface. The synthesized lateral heterojunction enables the reduced dimensions of Schottky barriers and enhanced carrier injection compared to counterparts composed of a vertical 3D metal contact. Furthermore, facile position-selected growth of PtTe 2 -MoS 2 MSJ arrays using conventional lithography can facilitate the design of device layouts with high processability, while providing low contact resistivity and ultrashort transfer length on wafer scales. The scaling of the dimensions of electronic components is essential to increase the density of devices in an integrated chip (IC) [1] , [2] . To fulfill industrial requirements, the transistors in ICs must have both ultrashort physical lengths of the gate ( L < ~12 nm) and contact ( L c , which should be smaller than the required tightest metal pitch, ∼ 16 nm) by 2034 [1] , [3] . In this respect, two-dimensional (2D) van der Waals (vdW) materials have emerged because of their higher carrier mobility and superior electrostatic controllability at the atomically thin limit [1] , [2] to achieve channel scaling for future nanoelectronics. However, fundamental limitations in producing ultra-scaled, low-resistance contact electrodes for 2D semiconductors (e.g., transition metal dichalcogenides (TMDs)) [2] , [4] using a conventional 3D metal contact limit the switching performance of transistor. For example, the deposition of the 3D metal contact onto 2D semiconducting TMDs typically yields a disorder-rich interface at the metal-semiconductor junction (MSJ), resulting in high contact resistance ( R c ) [2] , [4] . Furthermore, the resultant 3D/2D MSJs have inevitably long transfer length ( L T ) of charge carriers (e.g., L T > ∼ 50–200 nm) [5] , [6] , [7] , [8] , [9] , [10] , which leads to an exponential increase in R c with the reduction in the contact size if L c is smaller than L T (i.e., L c < L T ), prohibiting prospective contact scaling. To avoid the problems associated with conventional vertical contact, pioneering works on the use of edge-to-edge connected lateral 3D-2D (or 2D-2D) MSJs have been conducted [5] , [11] , [12] , [13] , [14] , [15] , [16] , [17] . It has a directly metalized junction with strong hybridization, and the absence of atomic discontinuities or defects at the lateral MSJs facilitates superior contact between the 2D semiconducting TMDs and metal electrodes (i.e., smaller R c ) [5] , [11] , [13] . Furthermore, using a lateral MSJ has a significant advantage in lowering the L T because the carriers are only injected through the few-atom-thick interface (i.e., L T decreases to a few nm). Thus, the lateral MSJ-based transistor performs excellently even if L c is reduced to the sub-nm range [5] . However, owing to the general thermal and chemical instability of TMDs, practical techniques for controlling heterogeneous integration are highly challenging. Only proof-of-concept has been demonstrated [5] , [11] , [13] , [14] , [15] , [16] , [17] , thereby failing to achieve high yield and high device density. For instance, obtaining edge contact by lithographic techniques requires that the 2D semiconductors be protected against oxidizing conditions using a passivation layer (e.g., hexagonal boron nitride) [11] , [13] , or in-situ etching prior to edge metallization [5] . Chemical vapor deposition (CVD) of TMD-based 2D-2D MSJ heterostructures lacks the control of spatial locations [12] , [14] , [15] , and their active layer is inevitably degraded by thermal budget effect because the synthesis of 2D semiconductors along the edge of 2D vdW metals are still at the embryonic stage of development. Although graphene has been widely studied for low-resistance contacts with 2D semiconductors [16] , [17] , the large lattice mismatch between graphene and the 2D semiconductor, along with the polymer-based residues incorporated into the assemblies during the graphene-transfer processes, commonly hinder the production of edge-contacted in-plane 2D-2D MSJs and limit the performance of the contacts [16] , [18] . Recent studies have demonstrated significant advances towards fabricating lateral 2D-2D MSJs using irregularly-formed flakes of 2D vdW metals, Mo 2 C and VS 2 [14] , [15] . However, for the approach to be practical and scalable, limitations in terms of the reproducibility of conformal MSJ patterns with sub-1-nm L T on a large scale and low R c through the suggested approach need to be addressed. Therefore, in the long term, it is vital to develop a groundbreaking technique for fabricating a 2D vdW metal with high stability and processability that can offer a substantial degree of freedom in the device architecture. Here, we demonstrate the formation of synthetic edge contacts consisting of metallic 2D vdW PtTe 2 crystals with high thermal stability and the facile position-selected growth of conformal lateral 2D-2D MSJ patterns using conventional lithography. We investigated the high thermal stability of PtTe 2 under ultrahigh vacuum (UHV) (which maintained its intrinsic surface property up to ∼ 825 °C) and succeeded in obtaining edge-directed PtTe 2 -MoS 2 lateral heterojunctions by using two-step CVD. The resultant epitaxially grown lateral MSJ sustained almost ideal stoichiometry without the development of thermally induced voids or the production of mixed alloys. The monolayer MoS 2 MSJ transistors with PtTe 2 edge contacts exhibited superior n -type carrier transport compared to those with 3D vertical contacts, attributed to both the reduced thermionic emission at the Schottky barrier and the lack of interfacial defects. Additionally, the position-controlled growth of PtTe 2 and subsequent chemical assembly to MoS 2 allowed us to obtain 2D TMD-based synthetic edge contact arrays on a large scale. The patterned MSJ showed ultralow contact resistivity (> 11.7 Ω·μm 2 ), which is almost one order of magnitude smaller than those of typical 3D top contact electrodes ( ∼ 10 3 to 10 5 Ω·μm 2 ), along with a significantly short L T ( ∼ 0.7 nm), indicating the potential of PtTe 2 for affording drastically miniaturized high-quality metal contacts to atomic transistors. Synthetic strategy for high-quality, edge-contact MSJ To produce electronic-grade edge contacts, we developed a synthesis method for lateral MSJs that ensures high-quality MoS 2 as a channel material. Many previous studies on lateral MSJs prepared using CVD rely on the growth of 2D metals after the preparation of 2D semiconductors because typical 2D semiconductors (e.g., WS 2 , MoSe 2 ) require a relatively high growth temperature ( ∼ 700–800 °C) compared to vdW metals (e.g., ∼ 600 °C for NbS 2 or VSe 2 ) [19] , [20] . However, this sequence for two-step CVD can thermal degrade 2D semiconductors, substantially lowering the performance of resultant device because of the increased chalcogen vacancies of the channel [21] . Instead, we developed a technique to create a 2D semiconductor (i.e., MoS 2 ) after preparing 2D metal (i.e., PtTe 2 ) to produce a high-quality semiconducting 2D sheet in the lateral MSJ (Fig. 1a, b ). Fig. 1: Formation of MoS 2 –PtTe 2 lateral heterostructure by two-step growth. a Schematic of the growth process for the PtTe 2 flakes at a growth temperature of 700 °C. b Schematic of the growth process of MoS 2 along the edge of PtTe 2 . The insets of ( a ) and ( b ) show the representative false-colored scanning electron microscopy (SEM) image of the synthesized PtTe 2 flakes and PtTe 2 -MoS 2 heterostructures on SiO 2 /Si substrate. c Raman spectra of multilayer PtTe 2 flakes displaying strong E g and A 1g signals (vertical dashed lines) without any substantial differences up to 900 °C annealing under UHV conditions. d Benchmark plots of metallic TMDs such as 1T’-WTe 2 [31] , [35] , 2H-NbSe 2 [32] , [37] , 1T’-MoTe 2 [33] , [38] , 1T-TaS 2 [36] , [39] , and 1T’-MoS 2 [34] with respect to the room-temperature electrical resistivity ( ρ ) and the endurance temperature, T , that the material can tolerate without structural degradation. The endurance T of the metallic TMDs were characterized under vacuum (solid) or Ar atmosphere (binned). e Confocal Raman spectrum captured at the heterojunction’s interface, PtTe 2 , and MoS 2 flakes. The vertical lines indicate E g and A 1g modes from PtTe 2 , and E 2g and A 1g modes from MoS 2 . f Atomic force microscopy (AFM) height profile along the red line displayed in the corresponding AFM image (inset, with a scale bar of 2.5 μm; the MoS 2 boundary is indicated as white dashed lines. ), indicating the synthesized MoS 2 forms a monolayer ( H ≈ 0.78 nm) while the PtTe 2 forms multiple layers (thickness, H ≈ 28 nm). g , h X-ray photoelectron spectroscopy (XPS) analysis of the PtTe 2 -MoS 2 heterostructure. For comparison, the spectra of bare MoS 2 grown independently on the substrate and those of Ti-deposited MoS 2 are displayed. The XPS profiles of the for Mo 3 d , and S 2 p regions are shown in ( g ) and ( h ), respectively. The XPS Mo 3 d 3/2 , Mo 3 d 5/2 , S 2 p 1/2 , and S 2 p 2/3 peaks are specified by dashed lines. i , j Transmission electron microscopy (TEM) investigations of the heterostructure consisting of a multilayer PtTe 2 with a monolayer MoS 2 . i Selected area electron diffraction (SAED) patterns of the MoS 2 -PtTe 2 heterostructure, showing the orientationally aligned (100) and (110) planes of each material, indicating the epitaxial growth of the MoS 2 . j (left) High-angle annular dark-field scanning-TEM (HAADF-STEM) image demonstrating the atomic arrangements at the MoS 2 -PtTe 2 heterojunction. (right) Schematic of the lateral heteroepitaxy aligned to the <100> direction. Full size image As an efficient edge contact metal for MoS 2 , we selected one of 2D metallic TMDs, PtTe 2 , because it exhibits many attractive features as potential n -type metal contacts for 2D semiconductors. For example, the theoretical work function (WF) of few-layered PtTe 2 (WF; ∼ 4.56–4.57 eV) [22] is one of the smallest among those reported for chemically synthesizable metallic TMDs [23] , [24] , [25] (Supplementary Fig. 1 ), and its electrical conductivity (>10 6 S/m) has shown to be the highest among 2D metals [26] , [27] . However, the simultaneous achievement of large-area production of high-quality stoichiometric, metallic TMD thin films with thermal stability remains challenging, mainly because of the difficulties in incorporating Te and low environmental stability during thermal CVD [28] , [29] . Furthermore, guaranteeing the thermal stability of the 2D metal is essential for our two-step CVD process because PtTe 2 must resist the thermal procedure required for synthesizing of MoS 2 while maintaining excellent quality. In this regard, no success has been achieved yet for 2D-2D lateral heterojunctions based on 2D tellurides. Since Te vacancies substantially reduce the Gibbs free energy for the adsorption of ambient gas and cause structural instability [30] , the growth of high-quality PtTe 2 is essential to ensure its stability to some extent. Thus, we synthesized the PtTe 2 crystals using the eutectic solidification method [26] , [31] , where the pre-deposited Pt precursor reacted with liquefied Te at 700 °C (Fig. 1a ). The resultant PtTe 2 formed single crystals with a highly stoichiometric nature (Supplementary Fig. 2 ). As our synthetic methods do not require an oxide precursor, no oxygen-metal bonds, which often become reactive sites and cause poor stability, were formed [32] . In addition, the PtTe 2 crystals maintained their high-quality structures with Te terminations even after exposure to air for up to ∼ 3 h, as indicated by TEM analysis (Supplementary Fig. 3 ). The WF of PtTe 2 ( ∼ 4.65 eV), characterized by ultraviolet photoelectron spectroscopy (UPS), was comparable to the computed value [22] (Supplementary Fig. 2h ), satisfying the basic requirement of an efficient n -type contact for the MoS 2 transistor, considering its band structure (Supplementary Fig. 1 ). To evaluate the thermal stability of the as-synthesized PtTe 2 , the crystal was annealed under UHV conditions ( ∼ 10 −10 Torr) at temperatures between T = 500–1000 °C for 1 h. The Raman spectra obtained are shown in Fig. 1c . The as-grown PtTe 2 and the UHV-annealed crystals heated to 900 °C showed comparable Raman in-plane E g ( ∼ 110 cm −1 ) and out-of-plane A 1g ( ∼ 156 cm −1 ) vibrational modes of PtTe 2 [27] (black dashed line in Fig. 1c ). Remarkably, only annealing above ∼ 1000 °C altered the peak positions and their intensities, demonstrating the high thermal stability of the PtTe 2 . The thermal stability is an intrinsic property independent of the thickness and degree of structure order, as evaluated by X-ray photoelectron spectrum (XPS) and UPS (Supplementary Fig. 4 ). The surface properties of PtTe 2 start to change above the T of ∼ 825 °C, which is far beyond the limitations of metallic TMDs (e.g., WTe 2 , MoTe 2 , TaS 2 , and 1 T’-MoS 2 ) measured under vacuum or in an Ar atmosphere [32] , [33] , [34] , [35] , [36] . In addition, low electrical resistivity of PtTe 2 ( ρ ≈ 0.37 mΩ·cm; Supplementary Fig. 5a, b ), even lower than other few-layered metallic TMDs [31] , [34] , [37] , [38] , [39] ( ρ ≈ 0.5–100 mΩ·cm), shows promise for a robust electrode that may prevent thermal stress as summarized in Fig. 1d . Following the synthesis of thermal-stable PtTe 2 multilayers, a monolayer of MoS 2 was formed laterally along the edge of the PtTe 2 by CVD at ∼ 700 °C (Fig. 1b ). Compared to the edge, the atomically pristine, dangling-bond-free surface of a 2D crystal typically possesses fewer surface defects and minimal MoS 2 nucleation. Density functional theory (DFT) simulations were performed to investigate the selective nucleation of MoS 2 on the edges of PtTe 2 . Adsorption energy calculations reveal that there was preferential adsorption and subsequent nucleation of MoS 2 at the PtTe 2 edge. For instance, the MoS 2 monomer exhibited a lower adsorption energy of −3.6 eV at the PtTe 2 edge compared to −2.7 eV on the PtTe 2 basal plane (Supplementary Fig. 6 ). These findings are consistent with those of previous reports on the two-step CVD of 2D heterostructures, where in the adsorption energy of 2D TMDs at the edge of a 2D crystal was lower than that on the 2D basal plane [19] , [40] . The low occurrence of MoS 2 nucleation on the PtTe 2 surface is attributed to the higher adsorption energy of MoS 2 nuclei on the basal plane. In our experiments, we significantly lowered the mass flux of precursors through the source-contact geometry and use of a MoO x thin-film precursor significantly reduced the opportunities for nucleation (Supplementary Note 1 ). The attachment of adatoms or atomic clusters of MoS 2 by heterogeneous nucleation was allowed only at the edge of PtTe 2 . The introduction of a higher mass flux would thus increase the possibility of producing more nucleations [41] and trigger the synthesis of randomly distributed multilayer MoS 2 on the structures. Attributed to the edge-mediated growth mode, the MoS 2 crystals were observed exclusively along the PtTe 2 edges as shown in false-colored scanning electron microscopy (SEM) images (inset of Fig. 1b and Supplementary Fig. 7 ). The Raman signals at the interface of MSJ demonstrated the strong signals of PtTe 2 without variation in positions, while the MoS 2 features of E 2g ( ∼ 384 cm −1 ) and A 1g ( ∼ 407 cm −1 ) modes also existed (Fig. 1e ). Most of the MoS 2 attached to PtTe 2 was a monolayer with a uniform thickness of ∼ 0.7 nm, as shown in the AFM image and height profile (Fig. 1f ). XPS analysis of the heterostructures was used to reveal the surface compositions and chemistries (Fig. 1g , h and Supplementary Fig. 8 ). The XPS spectra of the MoS 2 layer did not show a substantial peak shift compared to that of non-stitched bare flakes (green, Fig. 1g, h ). In comparison, the vertically deposited 3D metals on MoS 2 can induce surface defects [4] , [42] , that is, a non-stoichiometric layer (i.e., Mo x S y ) or alloys (i.e., Ti x S y ), as we experimentally demonstrated in the case of Ti/MoS 2 (gray, Fig. 1g ). Hence, the coincident binding energy of MoS 2 connected to PtTe 2 and that of the bare flakes suggests that the present growth mode conferred the intrinsic surface properties of the 2D semiconductor layer (i.e., MoS 2 ), as the MoS 2 layer was grown after preparing PtTe 2 . XPS analysis further revealed no noticeable change in the stoichiometry of PtTe 2 after thermal CVD for MoS 2 (at. % (Te/Pt) ≈ 1.80). This high stability of PtTe 2 during thermal CVD was also confirmed by SEM-EDS characterization (Supplementary Fig. 7d ). Pt and Te were the only two observed elements, and there were no apparent variations in their stoichiometry (that is, averaged at. % (Te/Pt) = 1.90 ± 0.06). In addition, we electrically characterized PtTe 2 to verify that the influence of the high-temperature process was negligible (Supplementary Fig. 5c, d ). The sustained low ρ (≈ 0.35 mΩ·cm) and the weak dependence on gate voltage ( V g ) imply that exposure to chemical species (MoO x and S) does not degrade PtTe 2 (Supplementary Fig. 5d ). Back-scattered SEM analysis did not show any traces of in-plane mixed alloying (Supplementary Fig. 7e–h ), further demonstrating the high stability of PtTe 2 . Structural analysis conducted using transmission electron microscopy (TEM) also confirmed the high quality of the PtTe 2 -MoS 2 lateral heterostructure (Fig. 1i, j , and Supplementary Figs. 9 – 11 ). We found that the MoS 2 monolayer grew epitaxially along the edge of PtTe 2 single crystal using the selected area electron diffraction (SAED) pattern (Fig. 1i ), indicated by the two aligned sets of hexagonal diffraction spots with six-fold symmetry reflecting the epitaxially aligned (110) and (100) lattice planes. Atomic-resolution analysis was performed using high-angle annular dark-field scanning-TEM (HAADF-STEM) (Fig. 1j ). The 2H-MoS 2 was atomically stitched to 1T-PtTe 2 without void-like defects. The high stoichiometry and compositional consistency of PtTe 2 were also confirmed by the STEM-EDS mapping and spectra (Supplementary Fig. 9a–f ). The electron energy loss spectroscopy (EELS) line scan further revealed the abrupt compositional change at the junction (Supplementary Fig. 9g–i ). Cross-sectional TEM analysis of synthetic MSJ also provided identical insight into the edge-to-edge connected structure, demonstrating in-plane epitaxial growth of MoS 2 and sharp interface at the junction (Supplementary Fig. 10 ). Remarkably, the absence of mixed or alloyed structures in the as-synthesized MSJ implies that our synthesis approach was successful. 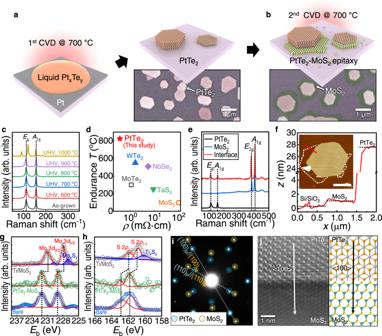Fig. 1: Formation of MoS2–PtTe2lateral heterostructure by two-step growth. aSchematic of the growth process for the PtTe2flakes at a growth temperature of 700 °C.bSchematic of the growth process of MoS2along the edge of PtTe2. The insets of (a) and (b) show the representative false-colored scanning electron microscopy (SEM) image of the synthesized PtTe2flakes and PtTe2-MoS2heterostructures on SiO2/Si substrate.cRaman spectra of multilayer PtTe2flakes displaying strongEgandA1gsignals (vertical dashed lines) without any substantial differences up to 900 °C annealing under UHV conditions.dBenchmark plots of metallic TMDs such as 1T’-WTe231,35, 2H-NbSe232,37, 1T’-MoTe233,38, 1T-TaS236,39, and 1T’-MoS234with respect to the room-temperature electrical resistivity (ρ) and the endurance temperature,T, that the material can tolerate without structural degradation. The enduranceTof the metallic TMDs were characterized under vacuum (solid) or Ar atmosphere (binned).eConfocal Raman spectrum captured at the heterojunction’s interface, PtTe2, and MoS2flakes. The vertical lines indicateEgandA1gmodes from PtTe2, andE2gandA1gmodes from MoS2.fAtomic force microscopy (AFM) height profile along the red line displayed in the corresponding AFM image (inset, with a scale bar of 2.5 μm; the MoS2boundary is indicated as white dashed lines.), indicating the synthesized MoS2forms a monolayer (H≈ 0.78 nm) while the PtTe2forms multiple layers (thickness,H≈ 28 nm).g,hX-ray photoelectron spectroscopy (XPS) analysis of the PtTe2-MoS2heterostructure. For comparison, the spectra of bare MoS2grown independently on the substrate and those of Ti-deposited MoS2are displayed. The XPS profiles of the for Mo 3d, and S 2pregions are shown in (g) and (h), respectively. The XPS Mo 3d3/2, Mo 3d5/2, S 2p1/2, and S 2p2/3peaks are specified by dashed lines.i,jTransmission electron microscopy (TEM) investigations of the heterostructure consisting of a multilayer PtTe2with a monolayer MoS2.iSelected area electron diffraction (SAED) patterns of the MoS2-PtTe2heterostructure, showing the orientationally aligned (100) and (110) planes of each material, indicating the epitaxial growth of the MoS2.j(left) High-angle annular dark-field scanning-TEM (HAADF-STEM) image demonstrating the atomic arrangements at the MoS2-PtTe2heterojunction. (right) Schematic of the lateral heteroepitaxy aligned to the <100> direction. This also demonstrates the merit of our approach compared to those adopted in previous studies [14] , [16] , [18] (as summarized in Supplementary Table 1 ). Interestingly, the high density of dangling bonds at the PtTe 2 edge generated several MoS 2 basal planes that were attached vertically to the edges of the PtTe 2 flakes (Supplementary Fig. 11 ). However, the vertical MoS 2 layers were relatively insignificant in the synthesized results because most MSJs possessed laterally stitched components without vertical structures. We performed DFT calculations to understand the formation mechanism of defect-free interface in the lateral PtTe 2 -MoS 2 MSJ (Supplementary Fig. 12 ). 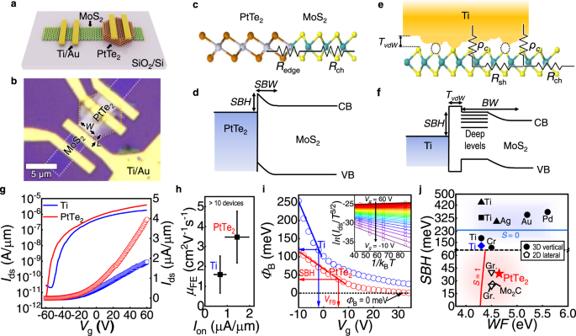Fig. 2: High performance of edge-contacted PtTe2-MoS2metal-semiconductor junction (MSJ) field-effect transistors (FETs). a–hMonolayer MoS2FETs with asymmetric carrier injection from PtTe2lateral epitaxial contact and from vertical Ti, characterized at room temperature.aSchematic and (b) optical microscopy image of a device with asymmetric Ti/Au and PtTe2electrodes contacted to a monolayer MoS2(white dashed lines) with a defined channel width (W) and length (L).c,eCross-sectional illustrations of resistance networks of monolayer MoS2-based MSJ with (c) atomically stitched PtTe2lateral contact and (e) top-contact with Ti/Au. Metallization of MoS2can degrade both the contact resistivity (ρc) and sheet resistance (Rsh) of MoS2. In contrast, the PtTe2-MoS2heterostructure has simpler resistance components, and the chemically derived edge resistance (Redge) is the only series resistance for the channel (Rch).d,fComparison of band alignments with different Schottky barrier heights (SBHs) and Schottky barrier width (SBW) with respect to the MoS2conduction band (CB) and valance band (VB) edges for (d) PtTe2-MoS2heterostructure and (f) conventional 3D metal-contacted MoS2. Tunneling barrier formed by vdW gap between Ti and MoS2(TvdW) and defect-induced deep levels are displayed in (f).gDrain current (Ids) as a function of gate voltage (Vg) for PtTe2-MoS2(red) and Ti/MoS2(blue) MSJ FETs on the logarithmic (lines; left) and linear (symbols; right) scales.hSummary of the field-effect mobility (μFE) and on-state current (Ion) of FETs with different carrier injections from PtTe2(red) and Ti (blue). The error bars indicate the standard deviations from each device set.i,jSBH of PtTe2-MoS2MSJ extracted using thermionic emission model.iCalculated thermionic barrier height of PtTe2-MoS2(red) and Ti/MoS2MSJ (blue) as a function ofVgshowing the low SBH of 38.5 meV at the flat band voltage. Inset: representative Arrhenius plot (ln(Ids/T3/2)vs. 1/kBT) of PtTe2-MoS2heterojunction with differentVg.jComparison of the SBH of few-layer MoS2based MSJ FETs with 3D top contacts (Ti47,48,49, Cr48, Ag49, Au48, and Pd48; solid) and with 2D lateral contacts (Mo2C15, and graphene16,17; open). The extracted SBHs of PtTe2-MoS2(red) and Ti/MoS2(blue) are indicated by colored symbols. Plots of the strength of Fermi-level pinning (S= |d(SBH)/d(WF)|) are shown as solid lines in order to compare the mechanism of formation of the SBHs. The calculated relative energies ( ΔE ) of the possible intermediates (i.e., MoO x and S adsorbents) attached to the PtTe 2 edge indicated the relative stability of each atomic structure during the epitaxial growth of MoS 2 (Supplementary Table 2 ). We found that reactive gas-phase S atoms were bound to MoO 3 precursor attached to the edge of PtTe 2 ( ΔE < −2.88 eV), and that O in MoO 3 tended to desorb as it reacted with additional S by forming SO 2 (g) because of the consequent exothermic processes. A similar repeated reduction process for MoO 3-x resulted in the formation of the most stable MoS 2 structure because of the substantial energy relative to the initial structure ( ΔE = −19.49 eV). Furthermore, each periodic interfacial cell comprised four PtTe 2 and five MoS 2 unit cells to minimize the lattice mismatch at the heterojunction (Supplementary Fig. 13 ). The lattice mismatch between PtTe 2 and MoS 2 was ∼ 18% when each unit cell of PtTe 2 was matched to a unit cell of MoS 2 in a one-to-one ratio according to the equation λ = (| a 1 − a 2 | )/ a 2 , where a 1 ( ∼ 3.25 ± 0.05 Å) and a 2 ( ∼ 3.96 ± 0.05 Å) are the in-plane lattice constants of MoS 2 [43] and PtTe 2 [44] , respectively (Supplementary Fig. 13a ). In comparison, adjusting the number of unit cells on the interface to a five-to-four ratio of MoS 2 and PtTe 2 resulted in a smaller mismatch between the materials ( ∼ 3%). STEM analysis also validated our heterostructure with consistently matched periodic cells along the <100> direction, indicating a (semi-)coherent interface (Supplementary Fig. 13b–d ). Given this smaller interfacial cell mismatch ( ∼ 3%), we calculated the most stable atomic structure for the heterostructure using DFT and the multicell model, as depicted in Supplementary Fig. 13b, c . The Pt-S and Mo-Te covalent bonds formed at the interface, resulted in strong orbital interactions between the atoms at the heterojunction. High-performance monolayer MoS 2 FETs with PtTe 2 edge contact We now shift our focus to the electrical characterization of the edge-contacted 2D-2D MSJ field-effect transistors (FETs). After the definition of MoS 2 channels by the reactive ion etching process, PtTe 2 -flake-connected MoS 2 MSJ FETs were fabricated by Ti/Au (10/70 nm) contact pad deposition on PtTe 2 . The Ti/Au layer was also deposited on the other side of the MoS 2 channel to produce an asymmetrical contacted MoS 2 channel with a fixed width ( W ) and length ( L ) for comparison with the MoS 2 -Ti vertical junction (Fig. 2a, b ). The gate bias was applied through the 300-nm-thick SiO 2 dielectric layer for this measurement. Because the reverse-biased contact (source) causes most of the voltage drop and dominates the transistor behavior in n -type MoS 2 MSJ FETs, the source (either Ti or PtTe 2 ) determines the performance of a FET with asymmetric contacts. This allows the electrical properties of the barrier to be systemically evaluated by controlling the interface [15] , [29] . We selected Ti as the counterpart to PtTe 2 because it is the most widely used contact and has a low WF of ∼ 4.33 eV [23] , which is even smaller than that of PtTe 2 ( ∼ 4.60-4.65 eV in Fig. 1g ). Fig. 2: High performance of edge-contacted PtTe 2 -MoS 2 metal-semiconductor junction (MSJ) field-effect transistors (FETs). a – h Monolayer MoS 2 FETs with asymmetric carrier injection from PtTe 2 lateral epitaxial contact and from vertical Ti, characterized at room temperature. a Schematic and ( b ) optical microscopy image of a device with asymmetric Ti/Au and PtTe 2 electrodes contacted to a monolayer MoS 2 (white dashed lines) with a defined channel width ( W ) and length ( L ). c , e Cross-sectional illustrations of resistance networks of monolayer MoS 2 -based MSJ with ( c ) atomically stitched PtTe 2 lateral contact and ( e ) top-contact with Ti/Au. Metallization of MoS 2 can degrade both the contact resistivity ( ρ c ) and sheet resistance ( R sh ) of MoS 2 . In contrast, the PtTe 2 -MoS 2 heterostructure has simpler resistance components, and the chemically derived edge resistance ( R edge ) is the only series resistance for the channel ( R ch ). d , f Comparison of band alignments with different Schottky barrier heights (SBHs) and Schottky barrier width (SBW) with respect to the MoS 2 conduction band (CB) and valance band (VB) edges for ( d ) PtTe 2 -MoS 2 heterostructure and ( f ) conventional 3D metal-contacted MoS 2 . Tunneling barrier formed by vdW gap between Ti and MoS 2 ( T vdW ) and defect-induced deep levels are displayed in ( f ). g Drain current ( I ds ) as a function of gate voltage ( V g ) for PtTe 2 -MoS 2 (red) and Ti/MoS 2 (blue) MSJ FETs on the logarithmic (lines; left) and linear (symbols; right) scales. h Summary of the field-effect mobility ( μ FE ) and on-state current ( I on ) of FETs with different carrier injections from PtTe 2 (red) and Ti (blue). The error bars indicate the standard deviations from each device set. i , j SBH of PtTe 2 -MoS 2 MSJ extracted using thermionic emission model. i Calculated thermionic barrier height of PtTe 2 -MoS 2 (red) and Ti/MoS 2 MSJ (blue) as a function of V g showing the low SBH of 38.5 meV at the flat band voltage. Inset: representative Arrhenius plot ( ln ( I ds / T 3/2 ) vs . 1/ k B T ) of PtTe 2 -MoS 2 heterojunction with different V g . j Comparison of the SBH of few-layer MoS 2 based MSJ FETs with 3D top contacts (Ti [47] , [48] , [49] , Cr [48] , Ag [49] , Au [48] , and Pd [48] ; solid) and with 2D lateral contacts (Mo 2 C [15] , and graphene [16] , [17] ; open). The extracted SBHs of PtTe 2 -MoS 2 (red) and Ti/MoS 2 (blue) are indicated by colored symbols. Plots of the strength of Fermi-level pinning ( S = |d(SBH)/d(WF)|) are shown as solid lines in order to compare the mechanism of formation of the SBHs. Full size image Figure 2g shows a representative transfer characterization ( I ds -V g ) of the MSJs where the electrons were injected from the PtTe 2 edge (red) and the vertical Ti contact (blue). In addition to the output curve (Supplementary Fig. 14a ), the on-state current ( I on ) of PtTe 2 -MoS 2 ( ∼ 4.0 μA/μm) was twice that of Ti-MoS 2 ( ∼ 1.8 μA/μm). The two-terminal field-effect mobility ( μ FE ) was also increased to ∼ 9.7 cm 2 V −1 s −1 by injection of charge carriers from PtTe 2 , compared to Ti ( ∼ 7.0 cm 2 V −1 s −1 ) for the same channel ( ∼ 3.5 ± 1.3 cm 2 V −1 s −1 and ∼ 1.6 ± 0.9 cm 2 V −1 s −1 on average for more than 10 devices with PtTe 2 and Ti asymmetric contacts, respectively; and the averaged values are demonstrated in Fig. 2h ). We found a slight negative shift of the turn-on voltage when the PtTe 2 source electrode was selected. This negative shift reflects the improved carrier injection from the contact [45] , [46] because the reduced R c and SBH caused the transistor easier to switch on (note that we could not observe an obvious doping effect on the in the XPS (Fig. 1g, h ) and Raman spectra (Fig. 1e ) after lateral epitaxy of PtTe 2 ). The performance enhancement was also confirmed for the MoS 2 FET with symmetric contact geometry (i.e., PtTe 2 -MoS 2 -PtTe 2 ; Supplementary Figs. 14b–e ). It showed a μ FE of ∼ 15.8 cm 2 V −1 s −1 , higher than those from asymmetrically contacted FET, which again verifies the influence of the resistance of the FET components related to Ti. High-energy deposition of a 3D metal typically degrades the surface of monolayer MoS 2 by forming sulfur vacancies and promoting atomic diffusion at MSJs [4] , [42] (i.e., forming interfacial defects of Ti/MoS 2 as shown in Fig. 1g, h ). These processes increase the R sh and contact resistivity ( ρ c ) by forming localized states as depicted in the contact components in Fig. 2e, f [29] , [47] , [48] , [49] . In addition, the established gap states can shift the charge neutrality, pinning the Fermi level to the mid-gap of MoS 2 , which can significantly impact the Schottky barrier height (SBH) [48] , [50] . According to Sze’s model [51] , the Fermi level pinning (FLP) strength increases with the density of interfacial traps ( D it ; Supplementary Fig. 15 and Supplementary Note 2 ); thus, the large D it in our Ti/MoS 2 MSJ FETs could induce strong FLP to the mid-gap states, and therefore resulted in a large SBH and lower thermionic emission efficiency over the SB. Furthermore, the top contact scheme has a long path for carrier transfer (e.g., wide width of the barriers, BW), leading to a larger R sh and ρ c . The vdW gap between the 3D metal and 2D semiconductor can also produce an additional tunnelling barrier ( T vdW ), although Ti/MoS 2 may possess a narrower T vdW than other 3D metals/MoS 2 because of the strong hybridization [2] , [42] . In contrast, the PtTe 2 -MoS 2 MSJ developed herein has a cleaner interface that prevents further metallization on the MoS 2 surface (i.e., absence of R sh ), leading to simple contact components only related to the edge (Fig. 2c, d ) [5] , [11] . The absence of T vdW and the reduced BW can improve carrier injection through the edge of PtTe 2 . Notably, despite the presence of a vdW gap between PtTe 2 and the metal contact pad (i.e., Ti/Au in Fig. 2a ), the contribution of R c in the Ti/PtTe 2 interface ( ∼ 0.12–0.23 kΩ·μm) of the MoS 2 -based MSJ system was insignificant ( ∼ 0.13%; Supplementary Fig. 16 ). 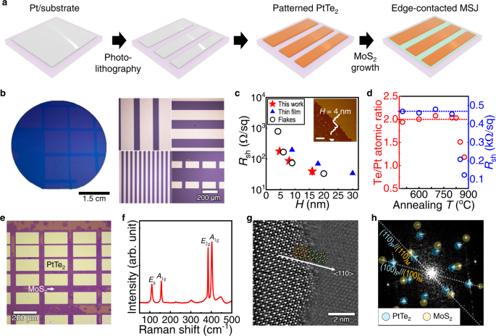Fig. 3: Wafer-scale growth of PtTe2patterns for synthetic edge contact arrays. aSchematic of procedure for realizing PtTe2-MoS2heterostructure arrays in a position-controllable manner, involving photolithography before the tellurization of Pt.bPhotograph image of as-grown large-scale PtTe2patterns on a 2-inch-scale SiO2/Si substrate (left), and representative OM images of the thin film captured on the left image (right).cSheet resistance (Rsh) of as-grown PtTe2thin film as a function of the film thickness (H), characterized by four-probe method.Rshvalues for high-quality PtTe2from previous reports27,53are displayed for comparison. The inset shows a representative AFM image of the as-grown thin film (scale bar: 1 μm).d(left) XPS-derived atomic ratio of the thin film, showing the nearly ideal stoichiometry of PtTe2(at. % (Te/Pt) ≈ 2; dashed red line) irrespective toTup to 825 °C, (right)Rshof thin films as a function of annealingT, withRsh~467 Ω/sq (forT= 500 °C) indicated with a blue dashed line.eRepresentative OM images of MoS2monolayer laterally contacted to the edge of polycrystalline PtTe2thin film patterns withH≈ 4 nm, in the form of fully stitched thin film depending on the growth conditions.fRepresentative Raman spectrum of PtTe2-MoS2heterostructure, showing strong signals of each material, e.g.,Eg(110.2 cm−1) andA1g(156.5 cm−1) peaks of PtTe2andE2g(384.5 cm−1) andA1g(402.3 cm−1) modes of MoS2.g,hTEM analysis of heterostructure with patterned PtTe2(H≈ 4 nm) and monolayer MoS2.gHAADF-STEM image of heterostructure showing epitaxially stitched PtTe2and MoS2without void-like defects along both surfaces.hDiffractogram corresponding to interface region, indicating orientationally aligned (100) and (110) planes in each atomic structure. Furthermore, the estimated R c of the Ti/PtTe 2 interface is almost the lowest value that can be obtained in a 3D metal/vdW metal interfacial system (Supplementary Table 3 ) and is even smaller than that obtained with the most widely used vdW metal (graphene). To gain insight into the physical characteristic associated with carrier transport through the barriers, the thermionic barrier heights ( ϕ B ) of the monolayer MoS 2 MSJ FETs with symmetric contacts of PtTe 2 and Ti were calculated by electrical characterization at low temperatures (Fig. 2i , j and Supplementary Fig. 17 ). This allowed us to extract the SBHs at the interface by fitting the Arrhenius plot to the thermionic emission model [48] : 
    I_ds=[AA^*T^3/2exp(-qϕ_B/k_BT)][exp(qV_ds/k_BT)-1]
 (1) Here, A is the junction area, and A * is the effective Richardson–Boltzmann constant. According to Eq. ( 1 ), the ϕ B can be extracted from the slope of the Arrhenius plot (inset of Fig. 2i ), resulting in ϕ B as a function of V g (Fig. 2i ). Interestingly, the ϕ B for PtTe 2 -contacted MSJ at the flat band voltage ( V FB ) was found to be a substantially small value of ∼ 35.9 ± 9.8 meV (average of four devices), where the primary carrier injection mechanism changed from the thermionic transport ( V g < V FB ) to tunneling ( V g > V FB , where the linear V g - ϕ B relation ends at this actual SBH). For V g values exceeding ∼ 30 V, ϕ B was negative, indicating tunneling-dominant electrical transport through the reduced SBW of the edge contact, which is difficult to achieve with the 3D metal contact owing to the wider BW and the presence of T vdW for the latter. For example, the SBW at the PtTe 2 -MoS 2 interface ( ∼ 0.94 nm) calculated using a classical model for Schottky diodes was smaller than that of the Ti/MoS 2 MSJ FETs ( ∼ 1.5 nm) (Supplementary Note 2 ). The extracted SBH ( ϕ B at V FB ) of ∼ 35.9 meV is considerably lower than that of the Ti/MoS 2 MSJ ( ∼ 125 meV) and almost one order of magnitude smaller than previously reported values for other 3D-metal/MoS 2 MSJ [47] , [48] , [49] (≈100–500 meV in Fig. 2j ). Deep energy level states were established primarily because the interface was degraded by penetration of the 3D metals into the MoS 2 band [29] , [47] , [48] , [49] (Fig. 2f ). Therefore, the SBH of the FETs with Ti contact was much higher than the ideal value calculated by applying the Schottky-Mott rule (e.g., SBH = WF – χ ≈ 0 meV, where χ is the electron affinity of monolayer MoS 2 (≈ 4.28 eV) [48] ). The deviation from the Schottky-Mott rule is substantial for 3D contacts; thus, SBHs cannot be effectively modulated by selecting the 3D metals, as the Fermi levels are pinned to the shifted charge-neutral level (CNL). The interface index, S (=|d(SBH)/d(WF)|), indicates the extent of the deviation [48] , which approaches zero for the 3D metal contacts (blue line in Fig. 2j ). This strong FLP ( S ≈ 0) agrees well with the theoretical model prediction [51] that the S value decreases with increasing interfacial defect density ( D it ≈ ∞). We found that the increase in D it due to the replacement of the edge PtTe 2 by a top Ti contact could approach ∼ 1.13 × 10 13 eV −1 cm −2 , and gave rise to a stronger FLP (Supplementary Fig. 15 and Supplementary Note 2 ). Compared with vertical 3D metal contacts, the synthetic edge contact can weaken the FLP because of the lowered dimensionality with fewer interfacial defects [10] , [13] , [50] , [52] Hence, the SBHs can follow the ideal Schottky-Mott limit to some extent ( S = 1; red line in Fig. 2j ), enabling the formation of tiny SBHs by using low-WF 2D metals. Furthermore, the impact of strong covalent bonds at the edge interface, which may result in a slight deviation from the perfect Schottky-Mott limit through the formation of a metal-induced gap state (MIGS) [13] , is less significant compared to that at the top contacts because of the 1D-like atomically thin interface (Supplementary Fig. 18 ). Accordingly, the SBH in all 2D lateral contacts (Mo 2 C [15] , and graphene [16] , [17] ) to few-layer MoS 2 MSJ FETs produced by CVD ( ∼ 26-45 meV) is much smaller than those of vertical 3D contacts (Fig. 2j ). Similarly, the FLP-free PtTe 2 edge interface allowed the achievement of a negligible SBH ( ∼ 35.9 meV) due to low WF of PtTe 2 ( ∼ 4.56 eV [22] ); this is one of the lowest WF values among 2D metals, as summarized in Supplementary Fig. 1 . This smaller SBH ( ∼ 35.9 meV) enabled improved thermionic emission and tunneling transport through the SB compared with the top-contact Ti/MoS 2 , which had a higher SBH ( ∼ 135 meV) and additional T vdW . A higher μ FE and on/off ratio was therefore achieved, as indicated by variation of carrier transport through the barriers with V g (Supplementary Fig. 19 ). Spatial arrangement of synthetic edge contacts As the ultimate approach for demonstrating the advantage of PtTe 2 with respect to material processing, we eventually controlled the spatial arrangement of the synthetic edge contacts at the microscopic level (Fig. 3a ). Powder-based tellurization was used to transform the Pt patterns prepared by conventional photolithography into PtTe 2 patterns at a low temperature of ∼ 400 °C (here, we used Pt instead of PtO x , which can assure high quality of the resultant PtTe 2 [32] ). Remarkably, the patterns were successfully manufactured on a 2-inch SiO 2 /Si wafer, which is vital for achieving scalable, mass production of PtTe 2 electrodes in any desired shapes (Fig. 3b ). The electrical characterization by the four-point probe method showed that the R sh of the as-synthesized PtTe 2 thin film was H -dependent due to the greater carrier scattering as H decreased (Fig. 3c ). The R sh values of the developed PtTe 2 samples were lower than those previously reported for CVD-grown films [53] , and comparable to those of single-crystalline flakes [27] , suggesting that the developed films are of high quality. We found that the XPS-extracted stoichiometries for 4-nm-thick PtTe 2 were almost perfect (at.% ratio of Te/Pt ≈ 2) independent on the thermal stress up to T ≈ 825 °C (Fig. 3d ), suggesting the high quality and thermal stability of the film (similar to the case for single crystals in Fig. 1 ). The R sh of the PtTe 2 thin film was also ∼ 450 Ω/sq for the samples annealed below 800 °C. However, it suddenly changed as T reached 850 °C ( R sh ≈ 208 Ω/sq), indicating the atomic displacements of Te (which begins to resemble the electrical properties of Pt, as noted in caption of Supplementary Fig. 4 ). Fig. 3: Wafer-scale growth of PtTe 2 patterns for synthetic edge contact arrays. a Schematic of procedure for realizing PtTe 2 -MoS 2 heterostructure arrays in a position-controllable manner, involving photolithography before the tellurization of Pt. b Photograph image of as-grown large-scale PtTe 2 patterns on a 2-inch-scale SiO 2 /Si substrate (left), and representative OM images of the thin film captured on the left image (right). c Sheet resistance ( R sh ) of as-grown PtTe 2 thin film as a function of the film thickness ( H ), characterized by four-probe method. R sh values for high-quality PtTe 2 from previous reports [27] , [53] are displayed for comparison. The inset shows a representative AFM image of the as-grown thin film (scale bar: 1 μm). d (left) XPS-derived atomic ratio of the thin film, showing the nearly ideal stoichiometry of PtTe 2 (at. % (Te/Pt) ≈ 2; dashed red line) irrespective to T up to 825 °C, (right) R sh of thin films as a function of annealing T , with R sh ~467 Ω/sq (for T = 500 °C) indicated with a blue dashed line. e Representative OM images of MoS 2 monolayer laterally contacted to the edge of polycrystalline PtTe 2 thin film patterns with H ≈ 4 nm, in the form of fully stitched thin film depending on the growth conditions. f Representative Raman spectrum of PtTe 2 -MoS 2 heterostructure, showing strong signals of each material, e.g., E g (110.2 cm −1 ) and A 1g (156.5 cm −1 ) peaks of PtTe 2 and E 2g (384.5 cm −1 ) and A 1g (402.3 cm −1 ) modes of MoS 2 . g , h TEM analysis of heterostructure with patterned PtTe 2 ( H ≈ 4 nm) and monolayer MoS 2 . g HAADF-STEM image of heterostructure showing epitaxially stitched PtTe 2 and MoS 2 without void-like defects along both surfaces. h Diffractogram corresponding to interface region, indicating orientationally aligned (100) and (110) planes in each atomic structure. Full size image Subsequent conducted thermal CVD of MoS 2 induces lateral epitaxy of monolayer MoS 2 from the edge of the arranged PtTe 2 patterns (Fig. 3e ). A key to achieving a fully stitched MoS 2 thin film between the PtTe 2 crystals (instead of small flakes) is the extension of the growth time while decreasing the deposition rate via delicate control of the atomic flux. A higher growth temperature (>730 °C) and extensive precursors (for MoO x and S) resulted in multilayer MoS 2 and alloyed MoS 2 /PtTe 2 structures due to the island growth mode, whereas the layer-by-layer growth mode was enabled by the opposite manner. Figure 3f shows a representative Raman spectrum of the heterojunction, which shows the vibrational modes of each layered crystal. The Raman peaks for MoS 2 in the flakes and at the interface did not differ significantly (e.g., the energy difference between E 2g and A 1g peaks ≈ 19 cm −1 ), suggesting the growth of monolayer MoS 2 . The HAADF-STEM image (Fig. 3g ) and its indexed diffractogram (Fig. 3h ) confirm epitaxial alignment between monolayer MoS 2 and PtTe 2 . The STEM(-EDS) and corresponding (inverse) FFT study also verified the formation of a well-stitched lateral heterojunction comprising high-quality atomic layers (Supplementary Fig. 20 ). We did not find any significant differences from the bare MoS 2 flake in the XPS characterization of MoS 2 grown along the PtTe 2 array (Supplementary Figs. 8c, d ). Transport in the edge-contacted PtTe 2 -MoS 2 MSJ FET arrays Arrays of FETs composed of edge-contacted MSJs patterns were fabricated and operated by using an Al 2 O 3 back-gate dielectric (Fig. 4a ). Analysis of the output and transfer characteristics (Fig. 4b, c ) showed that the monolayer MoS 2 FETs with PtTe 2 symmetric contacts exhibited a maximum μ FE value of ∼ 17.9 cm 2 V −1 s −1 ( ∼ 10.6 ± 2.9 cm 2 V −1 s −1 on average), I on of up to ∼ 3.4 μA/μm ( ∼ 2.3 ± 0.3 μA/μm) and I on / I off in the range of ∼ 10 7 to 10 8 , which are much higher than those fabricated using vertical Ti contacts on monolayer MoS 2 FETs with the same device geometries (channel L and W ). We repeatedly observed performance enhancement for a large number of devices (>15), where the averaged μ FE of the Ti/MoS 2 FET was ∼ 0.4 ± 0.3 cm 2 V −1 s −1 and the I on was ∼ 0.2 ± 0.1 μA/μm (Fig. 4d ). It is worthwhile to note that, considering their L and L T values, the μ FE value of the MoS 2 FETs with PtTe 2 edge contacts were either comparable or even higher than those of previously reported devices with various 3D edges (e.g., Sc [54] , Ti [50] , Au [10] , and Mn [13] ) or 2D lateral contacts (e.g., graphene (Gr.) [17] , [18] , [55] , [56] , and VS 2 [14] ) (Supplementary Figs. 21a–c ). Fig. 4: Electrical transport studies of the edge-contacted PtTe 2 -MoS 2 MSJ FETs array. a Schematic showing monolayer MoS 2 FETs with patterned PtTe 2 edge contacts (upper) and vertical Ti contacts (lower). The transfer length ( L T ) of the carrier and physically attained contact length ( L c ) are schematically demonstrated. b Representative I ds – V ds characteristics of monolayer MoS 2 FET with symmetric PtTe 2 and Ti contact electrodes depending on V g . c I ds – V g characteristics of corresponding devices on linear (symbols; right) and logarithmic scale (lines; left). d Average μ FE and I on of different FETs (>15 devices) contacted to PtTe 2 (red) or Ti (blue). The error bars indicate the standard deviations of each measurement set. e–g Determination of contact resistance ( R c ) of MSJs with different compositions using ( e , f ) TLM and ( g ) Y -function method. e TLM plot showing total resistance normalized by contact width ( RW ) as a function of L . The y -intercept y ields the 2 R c in units of Ω ∙ μm. Inset shows OM image of MoS 2 (purple-like) grown between edges of PtTe 2 patterned for TLM. (f) TLM-derived R c of PtTe 2 -MoS 2 MSJ FETs approaching ~168 ± 127 kΩ∙μm when the carrier density ( n 2D ) of ~9 × 10 12 cm −2 was largely induced by V g (red circles), which is significantly lower than that of Ti/MoS 2 (~4,285 ± 1,959 kΩ∙μm, blue squares). Solid lines specify curves fitted to the relation of R c depending on the n 2D ( R c ∝ n 2D −0.5 ) [2] . g Histograms of R c for PtTe 2 -MoS 2 (left) and Ti/MoS 2 MSJ FETs (right) extracted by the Y -function method (Supplementary Fig. 22 ). The lowest R c of PtTe 2 -MoS 2 obtained in this study was ~18.2 kΩ·μm and the average value reached ~113.0 ± 60.3 kΩ·μm. h Benchmark specific contact resistivity ( ρ c ) and L T of synthetic PtTe 2 contacts. The experimental data from MoS 2 FETs with lateral graphene contact (Gr. [16] , [55] ), 3D edge contacts (Ti [11] , Ni [5] , Au [10] , Sc [54] , and Mn [13] ), and top contacts (Ti [6] , [58] , Ni [59] , Au [7] , [10] , Ag [9] , and Mn [13] ) are demonstrated. The colored symbols are the extracted data for PtTe 2 (red stars) and Ti (blue circle) in this work. For fair comparison, the data are sorted by ρ c extraction methods, i.e., four-point probe (open), TLM (solid), and Y -function (half-open symbol). Full size image To determine whether the μ FE of a device was severely underestimated because of the contact property, we extracted the intrinsic mobility ( μ 0 ) of more than 30 different devices using the Y -function method (Supplementary Fig. 22 ). The μ 0 value is typically free from underestimation due to R c and provides a better indication of the intrinsic performance [11] , [55] , [57] . The averaged μ 0 value in our PtTe 2 -MoS 2 MSJ FETs was calculated to be ∼ 11.1 ± 4.5 cm 2 V −2 s −1 , which is almost comparable to the μ FE values ( ∼ 10.6 ± 2.9 cm 2 V −2 s −1 ) calculated using the transconductance ( g m = ∂ I ds / ∂ V g ). The insignificant difference between μ FE and μ 0 ( ∼ 4.5%) implies the presence of a minor contact barrier at the edge interface. Notably, by using a MSJ fabricated with transfer length method (TLM) patterns, we could determine the R c values of the monolayer MoS 2 FETs with PtTe 2 edge contact (Fig. 4e, f ). The TLM-driven R c reached ∼ 168 ± 127 kΩ·μm when a carrier density ( n 2D ) of ∼ 9 × 10 12 cm −2 was attained, which was largely induced by a V g of ∼ 19 V. This R c value is ∼ 25 times lower than that of its counterpart using Ti ( ∼ 4,285 ± 1,959 kΩ·μm) in Fig. 4f . We note that the demonstration of R c as a function of n 2D (= C ox ( V g - V th )/ q ) helps compare devices because n 2D includes information on the threshold voltage ( V th ) that can be varied by channel doping, the gate dielectric layer, and the interfacial trap density of the substrate [2] , [6] , [7] . The R c was also calculated using the Y -function method [11] , [55] , [57] (Fig. 4g and Supplementary Fig. 22 ), where the minimum R c of the device was ∼ 18 kΩ·μm ( ∼ 113 ± 60 kΩ·μm, on average) and ∼ 2,562 kΩ·μm ( ∼ 12,443 ± 8,406 kΩ·μm) for PtTe 2 -MoS 2 and Ti/MoS 2 , respectively. The average R c values were comparable to those extracted from the TLM, demonstrating the reliability of the characterization methods. The low R c obtained with PtTe 2 allowed the FETs to outperform the Ti/MoS 2 MSJ FETs (Fig. 4b–d ). The significantly low TLM-driven R c at the monolayer-thick interface (e.g., L T ≈ 0.7 nm) of the spatially-arranged PtTe 2 -MoS 2 MSJ suggests that the contact length ( L c ) can be further scaled without an increase in R c (Fig. 4h ), as an advantage. For 3D top contacts, R c increases as the L c decreases below the L T because current crowding becomes severe, according to the transmission line model [6] , [7] expressed as R c = \(\sqrt{{\rho }_{c}{R}_{{sh}}}\) cot( L c / L T ), where L T = \(\sqrt{{\rho }_{c}/{\rho }_{{sh}}}\) and ρ c (= R c ∙ L T ) is the specific contact resistivity (Supplementary Fig. 23 ). Thus, there have been tremendous efforts (i.e., insertion of an interlayer [6] , chemical doping [58] , [59] , and metal deposition under UHV conditions [7] ) to achieve immunity of R c to L c scaling by lowering both ρ c and L T (right panel in Fig. 4h ). However, the achievement of a small L T (< tens of nanometers) together with low ρ c is inherently challenging for 3D top contacts [8] , [9] , [10] . Instead, the edge contact can prospectively afford a negligible L T because carrier transport occurs strictly through the interface of the edge [5] , [11] , [13] as depicted in Fig. 4a . We summarize the device performances of MoS 2 FETs with 3D edge [5] , [10] , [11] , [13] , [50] , [54] or 2D lateral contacts [14] , [15] , [16] , [17] , [18] , [55] , [56] (Supplementary Table 5 ). Although a direct comparison of the contact properties with our device is inappropriate because of the differences in the L T values, MoS 2 channel thicknesses, and R c -extraction methods (see Supplementary Note 3 for more details), the developed PtTe 2 -MoS 2 MSJ had a significantly low ρ c (as low as ∼ 11.7 Ω·μm 2 ) and L T ≈ 0.7 nm, which is the lowest value among those reported for few-layer MoS 2 FETs with 2D lateral graphene [16] , [55] , or 3D edge (Ti [11] , Ni [5] , Au [10] , Sc [54] , and Mn [13] ) contacts (see the left panel in Fig. 4h and Supplementary Fig. 21d ), thus promising the realization of ultralow R c in L c -scaled transistors for next-generation 2D nanoelectronics. We propose that even further reduction of R c and SBH is possible in our PtTe 2 edge contact by achieving a multilayer lateral 2D-2D MSJ heterostructure, which can be attributed to the effectively screened interfacial traps from the substrates [13] , [60] , the downshift of the conduction band edge in multilayer MoS 2 [29] , and the weaker current crowding at the thicker heterointerface [6] , [7] , [8] , [9] , [10] , [13] . Moreover, the use of high- k dielectrics (e.g., HfO 2 , Sb 2 O 3 , SrTiO 3 ), passivation layers (e.g., BN), and top-gate structures, which were already applied in the previous edge-contact FETs [10] , [11] , [13] , [18] , [55] , can also improve the performance of our device, which can be due to the suppressed charge scattering and trapped states from surrounding disorders [60] . We report here a spatially-controlled, reproducible preparation of metallic vdW PtTe 2 crystals as a lateral edge contact with semiconducting monolayer MoS 2 . The high-quality stoichiometric PtTe 2 retained its surface properties even after CVD at the high temperature of ∼ 750 °C under UHV conditions. The edge of thermally stable PtTe 2 provides nucleation sites for the subsequently grown 2D semiconductor without noticeable thermal degradation, resulting in in-plane lateral MSJs without substantial interfacial issues such as alloying or void-like defects. Therefore, the PtTe 2 -MoS 2 MSJ may have a simple resistance network and displays superior n -type carrier transport through the short and narrow thermionic barriers, enabling the higher performance of the FET compared to that composed of vertical 3D contacts. This approach also provides a more scalable way to produce an arrangement of lateral heterostructures in a dimension-controlled manner, where the contact properties could be evaluated by using the TLM patterns consisting of the lateral MSJ. The substantially small contact resistivities achieved through the atomically thin edge suggest that the developed contact scheme has the potential for scaling the contact length for miniaturized 2D electronics. Our work on the synthesized edge-contact MSJ arrays offers benefits in terms of scalability for both material synthesis and device fabrication. The edge contact between 2D (or 3D) metals and 2D semiconductors should be developed and evaluated based on CVD-grown 2D layers to investigate its practical potential for semiconductor technology in the future. 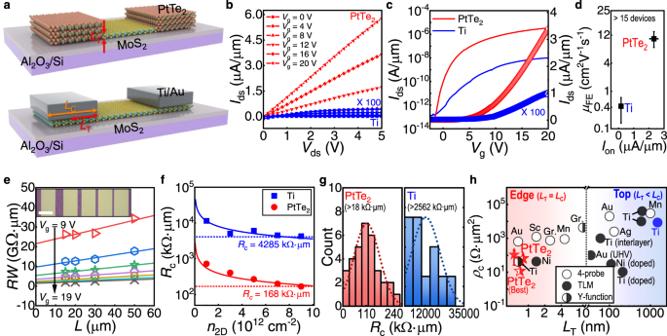Fig. 4: Electrical transport studies of the edge-contacted PtTe2-MoS2MSJ FETs array. aSchematic showing monolayer MoS2FETs with patterned PtTe2edge contacts (upper) and vertical Ti contacts (lower). The transfer length (LT) of the carrier and physically attained contact length (Lc) are schematically demonstrated.bRepresentativeIds–Vdscharacteristics of monolayer MoS2FET with symmetric PtTe2and Ti contact electrodes depending onVg.cIds–Vgcharacteristics of corresponding devices on linear (symbols; right) and logarithmic scale (lines; left).dAverageμFEandIonof different FETs (>15 devices) contacted to PtTe2(red) or Ti (blue). The error bars indicate the standard deviations of each measurement set.e–gDetermination of contact resistance (Rc) of MSJs with different compositions using (e,f) TLM and (g)Y-function method.eTLM plot showing total resistance normalized by contact width (RW) as a function ofL. They-interceptyields the 2Rcin units of Ω ∙ μm. Inset shows OM image of MoS2(purple-like) grown between edges of PtTe2patterned for TLM. (f) TLM-derivedRcof PtTe2-MoS2MSJ FETs approaching ~168 ± 127 kΩ∙μm when the carrier density (n2D) of ~9 × 1012cm−2was largely induced byVg(red circles), which is significantly lower than that of Ti/MoS2(~4,285 ± 1,959 kΩ∙μm, blue squares). Solid lines specify curves fitted to the relation ofRcdepending on then2D(Rc∝n2D−0.5)2.gHistograms ofRcfor PtTe2-MoS2(left) and Ti/MoS2MSJ FETs (right) extracted by theY-function method (Supplementary Fig.22). The lowestRcof PtTe2-MoS2obtained in this study was ~18.2 kΩ·μm and the average value reached ~113.0 ± 60.3 kΩ·μm.hBenchmark specific contact resistivity (ρc) andLTof synthetic PtTe2contacts. The experimental data from MoS2FETs with lateral graphene contact (Gr.16,55), 3D edge contacts (Ti11, Ni5, Au10, Sc54, and Mn13), and top contacts (Ti6,58, Ni59, Au7,10, Ag9, and Mn13) are demonstrated. The colored symbols are the extracted data for PtTe2(red stars) and Ti (blue circle) in this work. For fair comparison, the data are sorted byρcextraction methods, i.e., four-point probe (open), TLM (solid), andY-function (half-open symbol). However, almost all investigations on lateral MoS 2 -based MSJs have drawbacks in terms of reproducibility or the achievement of pure edge contact (Supplementary Table 4 ). In this regard, our strategy based on direct growth of a large-area 2D metal on a dielectric substrate followed by MoS 2 epitaxy has considerable advantages over other methods using 2D metals such as Mo 2 C [15] and graphene [16] , [17] , [18] , [55] , [56] , formed by mechanical exfoliation of single crystal and/or transfer of CVD-grown layers. More importantly, the realization of pure edge contacts with the L T reduced to ∼ 1 nm using graphene [16] , [17] , [18] , [55] , [56] or VS 2 [14] is highly challenging because of the inevitable laterally overlapped junction or alloyed structures. In addition, the construction of TLM patterns using a TMD-based synthetic edge contact provides assurance by permitting a better systematic analysis. Because of the complexity of realizing a lateral MSJ, it is difficult to achieve reproducible data from multiple devices and to perform statistical computations for R c [10] , [11] , [13] , [14] , [15] , [16] , [18] , [54] , [55] . Investigating R c of edge-contact MSJs using TLM pattern proves particularly challenging because of channel-to-channel variations and deficiencies in integration scalability. Many of the studies on lateral MSJ rely on the four-point measurement [10] , [13] , [14] , [15] , [16] , [18] , [54] or Y -function methods [11] , [55] for R c extraction, which can be inaccurate compared with the TLM (Supplementary Note 3 ). Therefore, together with the reproducibility of our 2D material system, the statistical analysis of the R c values extracted by TLM and the Y-function method in this study can provide better insights into the electrical features of 2D-2D edge contacts. Growth of PtTe 2 flakes The growth of multilayer PtTe 2 single crystals was conducted using a conventional horizontal furnace system, in which the Te-Pt precursors on a SiO 2 /Si substrate were placed inside the center of the chamber. To prepare the precursor sample, a Pt thin film precursor ( ∼ 2 nm, 99.9% purity pellet) was deposited using an e-beam evaporator (Temescal FC-2000), and then 0.1 g of Te powder was introduced manually to cover up the thin film. The reactant was then heated to ∼ 700 °C (at a heating rate of ∼ 50 °C/min) under a pressure of ∼ 0.1 Torr using H 2 (10 sccm) as the carrier gas. After maintaining a growth temperature of ∼ 700 °C for 1 min, the furnace was naturally cooled to room temperature. We succeeded in synthesizing PtTe 2 directly on top of the SiO 2 /Si substrate because the unreacted Te was vaporized and sucked out toward the vacuum pump. Preparation of patterned PtTe 2 thin films The pre-deposited, poly-crystalline Pt thin film ( ∼ 1 nm) on the SiO 2 /Si substrate and Te powder ( ∼ 0.1 g) inside a quartz boat were placed in a horizontal furnace ∼ 1 cm apart. Under low pressure (0.1 Torr) at ∼ 400 °C, the evaporated Te vapor reacts with the Pt precursor, resulting in a homogenous, uniform PtTe 2 layer with a thickness of ∼ 4 nm. The thickness of the as-grown thin film could be controlled by modulating the Pt precursor’s thickness. For position-controllability, the shape of any desired pattern was defined using photolithography (MIDAS MDA-400S) with a photoresist with an undercut profile (DPRi-1549), followed by Pt deposition and lift-off. Using the same method for thin films, the shaped Pt precursor could be tellurized, resulting in successful growth of the PtTe 2 patterns. Synthesis of MoS 2 along the edge of PtTe 2 The MoS 2 flakes were synthesized using MoO 3 thin film ( ∼ 1 nm-thick on a 1 cm 2 SiO 2 /Si substrate, evaporated using an e-beam evaporator) and S powder as precursors in atmospheric-pressure two-zone CVD with Ar/H 2 as the carrier gas. To promote the nucleation of MoS 2 , ∼ 1 μL of a 0.01 M NaCl promoter solution was pipetted on the corner of the oxide thin film on the substrate. Then, the NaCl solution was baked at ∼ 100 °C to evaporate the water entirely. The formerly prepared PtTe 2 multilayers on the substrate were placed face to face on top of the MoO 3 film prepared with NaCl. This metal oxide/PtTe 2 sample was placed at the center of the heat zone of the furnace, with the S-powder-containing boat loaded upstream of the CVD furnace. Under an Ar/H 2 ratio of 70/20 sccm, the system was steadily heated to ∼ 700 °C. At a growth temperature of ∼ 700 °C, S vapor was introduced because the powder was heated at ∼ 200 °C just before reaching the growth temperature and then maintained constantly for a growth time of ∼ 10 min. The as-synthesized PtTe 2 sample was stored in a chamber under UHV atmosphere ( ∼ 10 10 Torr) immediately after synthesis, and the air exposure time of PtTe 2 until the subsequent CVD process was <5 min. Structural characterization The morphological investigation was conducted using an SEM (Hitachi S-4800 or Su8220) equipped with high- and low-angle BSE detectors. Micro-Raman measurements were performed with a 532 nm laser (Thermo Scientific DXR2 Raman Microscope) configured for wavenumber precision of ≤0.066 cm −1 . XRD patterns were captured using a Bruker AXS D8 instrument with a Cu K α source. AFM images were recorded on a Bruker Dimension AFM operating in tapping mode. High-resolution STEM images, SAED patterns, EDS were obtained using an aberration-corrected FEI Titan 3 G2 60-300 equipped at an acceleration voltage of 200 kV. Noises of high-resolution STEM images were subtracted by Wiener filter. EELS was performed using a Gatan Quantum 965 dual EELS system with an energy resolution of 1.0 eV under an acceleration voltage of 200 kV. Specimen for cross-section TEM analysis were prepared by focused ion beam (FEI Helios Nanolab 450HP). XPS and UPS measurements were performed using an ESCALAB 250XI system (ThermoFisher K-alpha) equipped with an Al X-ray source under UHV conditions. The calibration of the XPS was performed by the alignment of the C 1 s spectrum (whose binding energy is 284.5 eV). DFT calculation We constructed a 4 × 4 × 1 PtTe 2 supercell with vacuum along the b and c directions to model a PtTe 2 single layer strap with an edge having 50% Te coverage. We performed geometry optimization based on DFT calculations using the supercell and the Vienna ab initio software packet [61] (VASP) code. We employed the projector-augmented-wave (PAW) method [62] and the Perdew-Burke-Enzerhof (PBE) functional [63] using a plane-wave basis set with an energy cutoff of 500 eV. The k-points were sampled using a 4 × 4 × 1 Monkhorst-Pack mesh [64] , and the spin-orbit coupling effect was also included. Electrical device fabrication and measurements To define the device channel, the shape of the channel layer was defined by e-beam lithography (NBL and NB3), and then a reactive ion etching process was conducted using SF 6 and O 2 plasma. The etched structures were transferred to a dielectric layer on highly p -doped Si, which can be used as the back-gate. For instance, the single-crystalline PtTe 2 -MoS 2 MSJ was transferred to a 300-nm-thick SiO 2 layer, whereas the conformally grown array was transferred to a 50-nm-thick Al 2 O 3 layer. The well-connected heterointerface between PtTe 2 and MoS 2 confirmed through TEM analysis (Figs. 1j and 3g ), proves that the wet transfer method utilizing a polymeric supporting layer did not affect the edge contact of the samples. The SiO 2 layer was dry-oxidized in a furnace (KHD-306) with ±3% uniformity, and the Al 2 O 3 dielectric layer was prepared by atomic layer deposition (Lucida, D100), being deposited within ±2% uniformity along the wafer. Ti/Au ( ∼ 10 and ∼ 70 nm, respectively) contacts and pads were then deposited using e-beam lithography and an e-beam evaporator. Electrical characterizations at different temperatures (138-300 K) were performed using a Keithley 4200-SCS detector in a cryogenic probe station (Lakeshore CRX-4K) under a high vacuum ( ∼ 10 −6 ). The μ FE of the FETs on the Al 2 O 3 dielectric insulator were determined by measuring the gate oxide capacitance per unit area ( C ox ) of Al 2 O 3 via C - V analysis of the metal-insulator-semiconductor structure (e.g., Pt/Al 2 O 3 / p ++ Si), where the DC voltage was swept from −5 to 10 V, while an AC voltage with an amplitude of ∼ 100 mV and frequency of ∼ 20 kHz was applied. The calculated C ox in the accumulation region was 0.164 ± 0.001 μF cm −2 (average of ten devices), which corresponds to an equivalent oxide thickness of ∼ 117.9 nm.